FoxO1 integrates direct and indirect effects of insulin on hepatic glucose production and glucose utilization FoxO proteins are major targets of insulin action. To better define the role of FoxO1 in mediating insulin effects in the liver, we generated liver-specific insulin receptor knockout (LIRKO) and IR/FoxO1 double knockout (LIRFKO) mice. Here we show that LIRKO mice are severely insulin resistant based on glucose, insulin and C-peptide levels, and glucose and insulin tolerance tests, and genetic deletion of hepatic FoxO1 reverses these effects. 13 C-glucose and insulin clamp studies indicate that regulation of both hepatic glucose production (HGP) and glucose utilization is impaired in LIRKO mice, and these defects are also restored in LIRFKO mice corresponding to changes in gene expression. We conclude that (1) inhibition of FoxO1 is critical for both direct (hepatic) and indirect effects of insulin on HGP and utilization, and (2) extrahepatic effects of insulin are sufficient to maintain normal whole-body and hepatic glucose metabolism when liver FoxO1 activity is disrupted. The liver is a key insulin target tissue for the control of glucose metabolism. For example, the effect of insulin to inhibit hepatic glucose production (HGP) is essential for maintenance of normal glucose homeostasis, and hepatic insulin resistance and impaired regulation of HGP contributes to hyperglycaemia in patients with diabetes [1] . FoxO transcription factors are major intracellular targets of insulin action and contribute to the regulation of gluconeogenic and glycolytic gene expression and nutrient metabolism in the liver [2] , [3] , [4] , [5] . Following the binding of insulin to the insulin receptor (IR), Akt is activated and phosphorylates FoxO proteins resulting in their translocation from the nucleus and sequestration in the cytoplasmic compartment, thereby suppressing effects of FoxO proteins on gene expression [6] . FoxO1 has been shown to interact directly with DNA binding sites in the promoter region of several genes involved in gluconeogenesis [7] , [8] and promotes glucose production both in isolated hepatocytes [9] and in transgenic mouse models [2] , [10] . Conversely, disruption of FoxO1 restores glucose tolerance to mice in which downstream targets of the insulin signalling pathway have been knocked out in a liver-specific manner [11] , [12] . These observations support the concept that insulin-mediated suppression of liver FoxO1 activity plays a critical role in glucose homeostasis and is crucial for inhibition of HGP by insulin. A recent report by Lu, et al. [12] indicated that disruption of FoxO1 in the liver restores the ability of insulin to suppress HGP even in mice in which Akt signalling has been disrupted. This finding has suggested that FoxO1 not only mediates metabolic consequences of liver insulin resistance, but also that hepatic glucose metabolism can be controlled via other insulin signalling pathways when the activity of FoxO1 has been disrupted [13] . However, it is not clear if this requires other direct effects of insulin acting through the IR in the liver, or whether indirect effects of insulin acting through non-hepatic target tissues (for example, brain, adipose tissue) can effectively control HGP and restore glucose homeostasis in animals that lack the hepatic IR, so long as FoxO1 is no longer active in the liver. To address this question and to more fully explore the role of FoxO1 in mediating the effects of hepatic IR signalling on glucose homeostasis, we compared the glucose metabolic phenotype of liver-specific IR knockout (LIRKO) mice with that of IR/FoxO1 double knockout (LIRFKO) mice. Our results indicate that liver FoxO1 is required for systemic glucose intolerance in hepatic insulin resistance [12] , [14] and provide evidence that insulin can effectively regulate both HGP and hepatic glucose utilization (HGU) through extrahepatic mechanisms when IR signalling has been disrupted and the function of FoxO1 is suppressed in the liver. Thus, hepatic (but not extrahepatic) insulin signalling appears to be entirely dispensable for the regulation of HGP and normal glucose homeostasis in LIRFKO mice, and regulation of FoxO1 function in the liver is essential for integrating direct and indirect effects of insulin on HGP and utilization. Phenotype validation Western blotting confirmed targeted disruption of IR in the liver of LIRKO mice, and deletion of both IR and FoxO1 in the liver of LIRFKO mice ( Fig. 1a ). Insulin-stimulated phosphorylation of hepatic Akt and FoxO1 was disrupted in both LIRKO and LIRFKO mice ( Fig. 1a ), demonstrating that insulin is not able to activate Akt signalling pathway in the absence of the hepatic IR ( Fig. 1a ). We also confirmed that the expression of the IGF-I receptor, which can interact with insulin at reduced affinity but is not expressed in normal adult hepatocytes [15] , is not increased in the liver of LIRKO or LIRFKO mice ( Fig. 1b ). Body fat mass was modestly increased in LIRKO mice compared with LIRFKO mice and floxed controls ( Fig. 1c ). However, neither body weight nor lean body mass differed significantly between genotypes ( Fig. 1c ). Liver weight was reduced by ∼ 25% in LIRKO mice compared with IR fl/fl (IR floxed) controls, and this effect was partially reversed (20% reduction) in LIRFKO mice ( Fig. 1d ). In contrast, glycogen content was decreased by ∼ 40% in both LIRKO and LIRFKO compared with control mice ( Fig. 1d ). Histological analysis of the liver revealed occasional hepatocellular atypia ( Fig. 1e ) and altered mitochondrial morphology ( Fig. 1f ) in LIRKO mice, consistent with previous studies [14] , but these changes were not detected in LIRFKO mice. Disrupting FoxO1, therefore, partially restores reduced liver weight, has a limited effect on glycogen content and rescues the abnormal cellular and mitochondrial morphology characteristic of liver-specific IR knockout mice. 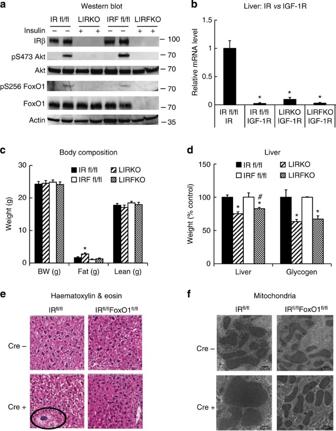Figure 1: Liver-specific insulin receptor knockout (LIRKO) and IR/FoxO1 double knockout (LIRFKO) mice. (a) Western blot. IR floxed (IR fl/fl), LIRKO, IR/FoxO1 floxed (IRF fl/fl) and LIRFKO mice were fasted for 4 h, then treated with insulin (10 U kg−1i.p.) and killed 10 min later. Liver lysates were analysed by western blotting with specific antibodies against the insulin receptor β subunit (IRβ), serine 473-phosphorylated Akt, total Akt, serine 256-phosphorylated FoxO1, total FoxO1 or actin, as shown. Molecular weight markers are shown for each protein. (b) Insulin receptor (IR) and insulin-like growth factor-1 receptor (IGF-1R) expression in liver. IR and IGF-1R expression was measured by quantitative PCR in liver from freely fed IR fl/fl (N=5), LIRKO (N=4) and LIRFKO (N=4) mice and expressed relative to IR mRNA levels in IR fl/fl mice. (c) Body weight and body composition. Body weight and body fat and lean mass (by NMR) are shown for 8-week-old male freely feeding IR floxed (solid bar,N=10), LIRKO (hatched bar,N=5), IR/FoxO1 floxed (open bar,N=13) and LIRFKO (cross-hatched bar,N=9) mice. (d) Liver weight and glycogen content. Liver weight and glycogen content were measured in tissues collected 6 h after refeding in IR floxed (N=12), LIRKO (N=10), IR/FoxO1 floxed (N=7) and LIRFKO (N=8) mice. Left. Liver weight adjusted for total body weight is expressed relative to floxed littermate controls. Right. Liver glycogen per mg protein is expressed relative to floxed littermate controls. (e) Haematoxylin and eosin stain. Liver was fixed in paraformaldehyde and embedded in paraffin prior to sectioning and staining, and slides were visualized by scanning at × 200 (Aperio Scanscope CS). Cellular atypia present in LIRKO liver is noted (circle). (f) Electron microscopy. Tissues were fixed with glutaraldehyde–paraformaldehyde and prepared for electron microscopy as described in Methods. The solid line in the lower right hand corner measures 500 nM. Results inFig. 1b–dare presented as the mean and s.e.m. Statistical significance (*P<0.05 versus IR floxed mice and#P<0.05, LIRFKO versus LIRKO mice) was determined by one-way analysis of variance and Fisher’spost-hoctest. Figure 1: Liver-specific insulin receptor knockout (LIRKO) and IR/FoxO1 double knockout (LIRFKO) mice. ( a ) Western blot. IR floxed (IR fl/fl), LIRKO, IR/FoxO1 floxed (IRF fl/fl) and LIRFKO mice were fasted for 4 h, then treated with insulin (10 U kg −1 i.p.) and killed 10 min later. Liver lysates were analysed by western blotting with specific antibodies against the insulin receptor β subunit (IRβ), serine 473-phosphorylated Akt, total Akt, serine 256-phosphorylated FoxO1, total FoxO1 or actin, as shown. Molecular weight markers are shown for each protein. ( b ) Insulin receptor (IR) and insulin-like growth factor-1 receptor (IGF-1R) expression in liver. IR and IGF-1R expression was measured by quantitative PCR in liver from freely fed IR fl/fl ( N= 5), LIRKO ( N= 4) and LIRFKO ( N= 4) mice and expressed relative to IR mRNA levels in IR fl/fl mice. ( c ) Body weight and body composition. Body weight and body fat and lean mass (by NMR) are shown for 8-week-old male freely feeding IR floxed (solid bar, N= 10), LIRKO (hatched bar, N= 5), IR/FoxO1 floxed (open bar, N= 13) and LIRFKO (cross-hatched bar, N= 9) mice. ( d ) Liver weight and glycogen content. Liver weight and glycogen content were measured in tissues collected 6 h after refeding in IR floxed ( N= 12), LIRKO ( N= 10), IR/FoxO1 floxed ( N= 7) and LIRFKO ( N= 8) mice. Left. Liver weight adjusted for total body weight is expressed relative to floxed littermate controls. Right. Liver glycogen per mg protein is expressed relative to floxed littermate controls. ( e ) Haematoxylin and eosin stain. Liver was fixed in paraformaldehyde and embedded in paraffin prior to sectioning and staining, and slides were visualized by scanning at × 200 (Aperio Scanscope CS). Cellular atypia present in LIRKO liver is noted (circle). ( f ) Electron microscopy. Tissues were fixed with glutaraldehyde–paraformaldehyde and prepared for electron microscopy as described in Methods. The solid line in the lower right hand corner measures 500 nM. Results in Fig. 1b–d are presented as the mean and s.e.m. Statistical significance (* P <0.05 versus IR floxed mice and # P <0.05, LIRFKO versus LIRKO mice) was determined by one-way analysis of variance and Fisher’s post-hoc test. Full size image Glucose tolerance and insulin sensitivity Fasting blood glucose levels were similar in LIRKO and LIRFKO mice, and 6-h refed glucose levels were only modestly increased in LIRKO mice versus IR floxed control and LIRFKO mice ( Fig. 2a ). In contrast, fasting and refed insulin levels were increased by ∼ 10-fold in LIRKO mice compared with controls and this hyperinsulinemia was fully reversed in LIRFKO mice ( Fig. 2b ). C-peptide levels also were increased in LIRKO, but not in LIRFKO mice ( Fig. 2c ), consistent with increased insulin secretion in LIRKO versus LIRFKO mice. In contrast, the C-peptide/insulin ratio, which reflects insulin clearance, was reduced in both LIRKO and LIRFKO mice compared with floxed controls ( Fig. 2d ), consistent with the absence of hepatic IR in both genotypes. Together, these findings indicate that the hyperinsulinemia of LIRKO mice results primarily from insulin hypersecretion rather than from differences in insulin clearance, which also is affected in LIRFKO mice. Consistent with this interpretation, islet mass was increased by approximately threefold in LIRKO versus IR floxed control mice ( Fig. 2e ), similar to previous studies [16] , and this effect was also reversed by liver-specific FoxO1 deletion ( Fig. 2e ). 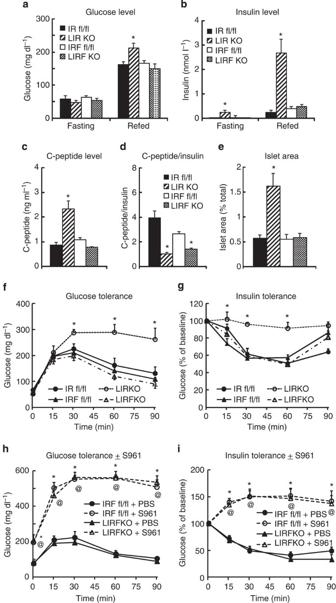Figure 2: Glucose and insulin levels, islet mass and glucose and insulin tolerance. Mice were fasted for 18 h overnight and then refed or left to fast until sacrifice 6 h later. Circulating levels of (a) glucose (IR floxed,N=17 fasting,N=17 refed; LIRKO,N=17 fasting, 18 refed; IR/FoxO1 floxed,N=16 fasting, 20 refed; LIRFKO,N=16 fasting, 20 refed) and (b) insulin (IR floxed,N=5 fasting, 6 refed; LIRKO,N=6 fasting, 6 refed; IR/FoxO1 floxed,N=4 fasting, 4 refed; LIRFKO,N=5 fasting, 4 refed) are shown. (c) C-peptide. Serum levels of C-peptide were measured in refed IR floxed (N=6), LIRKO (N=6), IR/FoxO1 floxed (N=6) and LIRFKO (N=4) mice. (d) C-peptide/insulin ratio. The ratio of C-peptide to insulin was calculated to evaluate effects on insulin clearance in IR floxed (N=6), LIRKO (N=6), IR/FoxO1 floxed (N=4) and LIRFKO (N=5) mice. (e) Islet mass. Islet and total pancreatic cross-sectional area were determined in scanned images and islet area expressed relative to total pancreatic area is shown for IR floxed (N=6), LIRKO (N=6), IR/FoxO1 floxed (N=6) and LIRFKO (N=6) mice. (f) Glucose tolerance. IR floxed (solid circle, solid line,N=6), LIRKO (open circle, dashed line,N=5), IR/FoxO1 floxed (solid triangle, solid line,N=4) and LIRFKO (open triangle, dot-dash line,N=5) mice were fasted 18 h overnight and glucose levels in tail blood were measured at baseline and 15, 30, 60 and 90 min after treatment with dextrose (2 g kg−1i.p.). (g) Insulin tolerance. IR floxed (solid circle, solid line,N=6), LIRKO (open circle, dashed line,N=5), IR/FoxO1 floxed (solid triangle, solid line,N=8) and LIRFKO (open triangle, dot-dash line,N=7) were fasted for 3 h and glucose levels were measured at baseline and 15, 30, 60 and 90 min after treatment with insulin (1 U kg−1i.p.). (h) Glucose tolerance w/wo S961 treatment. Overnight fasted IR/FoxO1 floxed and LIRFKO mice (N=5–7 per group) were treated with S961 in PBS or PBS alone 30 min prior to treatment with dextrose (2 g kg−1i.p.;t=0). (i) Insulin tolerance w/wo S961 treatment. IR/FoxO1 floxed and LIRFKO mice (N=5–7 per group) were fasted for 3 h then treated with S961 30 min before treatment with insulin (t=0). Results are presented as the mean and s.e.m. in each figure, and statistical significance (*P<0.05 versus IR floxed control, and@P<0.05 LIRFKO versus IRF floxed mice) was determined by one-way analysis of variance and Fisher’spost-hoctest. Figure 2: Glucose and insulin levels, islet mass and glucose and insulin tolerance. Mice were fasted for 18 h overnight and then refed or left to fast until sacrifice 6 h later. Circulating levels of ( a ) glucose (IR floxed, N= 17 fasting, N= 17 refed; LIRKO, N= 17 fasting, 18 refed; IR/FoxO1 floxed, N= 16 fasting, 20 refed; LIRFKO, N= 16 fasting, 20 refed) and ( b ) insulin (IR floxed, N= 5 fasting, 6 refed; LIRKO, N= 6 fasting, 6 refed; IR/FoxO1 floxed, N= 4 fasting, 4 refed; LIRFKO, N= 5 fasting, 4 refed) are shown. ( c ) C-peptide. Serum levels of C-peptide were measured in refed IR floxed ( N= 6), LIRKO ( N= 6), IR/FoxO1 floxed ( N= 6) and LIRFKO ( N= 4) mice. ( d ) C-peptide/insulin ratio. The ratio of C-peptide to insulin was calculated to evaluate effects on insulin clearance in IR floxed ( N= 6), LIRKO ( N= 6), IR/FoxO1 floxed ( N= 4) and LIRFKO ( N= 5) mice. ( e ) Islet mass. Islet and total pancreatic cross-sectional area were determined in scanned images and islet area expressed relative to total pancreatic area is shown for IR floxed ( N= 6), LIRKO ( N= 6), IR/FoxO1 floxed ( N= 6) and LIRFKO ( N= 6) mice. ( f ) Glucose tolerance. IR floxed (solid circle, solid line, N= 6), LIRKO (open circle, dashed line, N= 5), IR/FoxO1 floxed (solid triangle, solid line, N= 4) and LIRFKO (open triangle, dot-dash line, N= 5) mice were fasted 18 h overnight and glucose levels in tail blood were measured at baseline and 15, 30, 60 and 90 min after treatment with dextrose (2 g kg −1 i.p.). ( g ) Insulin tolerance. IR floxed (solid circle, solid line, N= 6), LIRKO (open circle, dashed line, N= 5), IR/FoxO1 floxed (solid triangle, solid line, N= 8) and LIRFKO (open triangle, dot-dash line, N= 7) were fasted for 3 h and glucose levels were measured at baseline and 15, 30, 60 and 90 min after treatment with insulin (1 U kg −1 i.p.). ( h ) Glucose tolerance w/wo S961 treatment. Overnight fasted IR/FoxO1 floxed and LIRFKO mice ( N= 5–7 per group) were treated with S961 in PBS or PBS alone 30 min prior to treatment with dextrose (2 g kg −1 i.p. ; t =0). ( i ) Insulin tolerance w/wo S961 treatment. IR/FoxO1 floxed and LIRFKO mice ( N= 5–7 per group) were fasted for 3 h then treated with S961 30 min before treatment with insulin ( t =0). Results are presented as the mean and s.e.m. in each figure, and statistical significance (* P <0.05 versus IR floxed control, and @ P <0.05 LIRFKO versus IRF floxed mice) was determined by one-way analysis of variance and Fisher’s post-hoc test. Full size image Glucose tolerance ( Fig. 2f ) and insulin tolerance ( Fig. 2g ) were markedly impaired in LIRKO mice, consistent with previous studies [16] , and both defects were fully rescued by hepatic FoxO1 deletion ( Fig. 2f,g ). Thus, hepatic FoxO1 is required for the impaired glucose tolerance and insulin resistance phenotype in LIRKO mice. These results indicate that hepatic IR signalling is not required for normal glucose homeostasis when the expression of FoxO1 is disrupted in the liver. At the same time, treatment with S961, a highly specific IR antagonist [17] , disrupted glucose tolerance ( Fig. 2h ) and glucose lowering effects of insulin ( Fig. 2i ) in LIRFKO mice ( Fig. 2h,i , respectively), indicating that extrahepatic IR-mediated effects of insulin are required for the restoration of both glucose tolerance and glucose lowering effects of insulin when both FoxO1 and IR have been disrupted in the liver. Glucose disposal and hepatic gene expression To explore the mechanisms whereby disrupting hepatic FoxO1 normalizes glucose homeostasis in LIRKO mice, we performed additional glucose tolerance studies using uniformly labelled 13 C-glucose (2 g kg −1 i.p.). We examined circulating levels of endogenous ( 12 C-) and exogenous ( 13 C-) glucose 60 min after 13 C-glucose injection, a time point when total blood glucose levels were approximately twofold higher in LIRKO compared with either IR floxed or LIRFKO mice ( Fig. 3a ). As shown in Fig. 3b , 12 C-glucose levels were increased by ∼ 50% in LIRKO relative to IR floxed and LIRFKO mice. Thus, impairment of endogenous glucose metabolism partially accounted for increased total glucose levels in LIRKO mice at this time point. Levels of uniformly labelled 13 C-glucose in LIRKO mice were 2- and 2.8-fold higher compared with IR floxed control and LIRFKO mice, respectively, indicating that (1) disposal of exogenous 13 C-glucose is significantly reduced in LIRKO mice, and (2) disrupting FoxO1 in the liver is sufficient to restore the disposal of an exogenous glucose load in the absence of the hepatic IR. The reduction in exogenous 13 C-glucose disposal in LIRKO mice was not due soley to increased endogenous 12 C-glucose production, since the enrichment of 13 C-glucose relative to 12 C-glucose was increased (and not decreased) in LIRKO mice compared with IR floxed and LIRFKO mice ( Fig. 3b ). 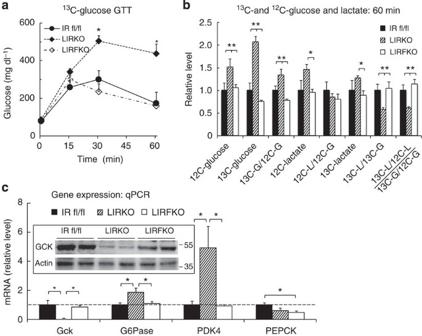Figure 3:13C-glucose tolerance and gene regulation. (a) Glucose levels. IR floxed (solid circles, solid line,N=9), LIRKO (solid diamond, dot-dashed line,N=13) and LIRFKO mice (open diamond, dashed line,N=10) were fasted for 18 h overnight, and then treated with13C-glucose (2 g kg−1i.p.). Blood glucose levels were measured at the indicated time points, and mice were killed at 60 min for analysis of glucose and lactate isotopomer levels and hepatic gene expression. (b)13C- and12C-glucose and lactate levels. Plasma12C- and13C-glucose and lactate levels were measured in IR floxed (N=4), LIRKO (N=6) and LIRFKO (N=4). Results for levels and calculated ratios were expressed relative to IR floxed mice. (c) Gene expression: quantitative PCR. Glucokinase (Gck), glucose-6 phosphatase (G6Pase), pyruvate dehydrogenase kinase 4 (PDK4) and phosphoenolpyruvate carboxykinase (PEPCK) mRNA levels were measured in liver collected 60 min post glucose by quantitative PCR and expressed relative to IR floxed mice (N=8, 8 and 8 for IR floxed, LIRKO and LIRFKO mice, respectively). *P<0.05 by one-way analysis of variance and Fisher’spost-hoctest. Figure 3: 13 C-glucose tolerance and gene regulation. ( a ) Glucose levels. IR floxed (solid circles, solid line, N= 9), LIRKO (solid diamond, dot-dashed line, N= 13) and LIRFKO mice (open diamond, dashed line, N= 10) were fasted for 18 h overnight, and then treated with 13 C-glucose (2 g kg −1 i.p.). Blood glucose levels were measured at the indicated time points, and mice were killed at 60 min for analysis of glucose and lactate isotopomer levels and hepatic gene expression. ( b ) 13 C- and 12 C-glucose and lactate levels. Plasma 12 C- and 13 C-glucose and lactate levels were measured in IR floxed ( N= 4), LIRKO ( N= 6) and LIRFKO ( N= 4). Results for levels and calculated ratios were expressed relative to IR floxed mice. ( c ) Gene expression: quantitative PCR. Glucokinase (Gck), glucose-6 phosphatase (G6Pase), pyruvate dehydrogenase kinase 4 (PDK4) and phosphoenolpyruvate carboxykinase (PEPCK) mRNA levels were measured in liver collected 60 min post glucose by quantitative PCR and expressed relative to IR floxed mice ( N= 8, 8 and 8 for IR floxed, LIRKO and LIRFKO mice, respectively). * P <0.05 by one-way analysis of variance and Fisher’s post-hoc test. Full size image We also measured circulating levels of 12 C-lactate and uniformly labelled 13 C-lactate 60 min after the administration of the 13 C-glucose load. Circulating levels of 12 C-lactate, which is produced from multiple substrates, including endogenous glucose, glycogen stores and pyruvate derived from amino acids, were increased in LIRKO mice by ∼ 50% compared with other genotypes ( Fig. 3b ), an effect that was proportional to the increase of circulating 12 C-glucose levels ( Fig. 3b ). Although circulating levels of 13 C-lactate (which is produced only by metabolism of exogenous 13 C-glucose and is therefore more directly related to disposal of a glucose load) also tended to be modestly elevated in LIRKO versus IR floxed and LIRFKO mice, the ratio of 13 C-lactate to 13 C-glucose levels ( 13 C-lactate/ 13 C-glucose) was reduced by ∼ 40% in LIRKO compared with both IR floxed and LIRFKO mice. Further, 13 C-lactate enrichment ( 13 C-lactate/ 12 C-lactate) relative to glucose enrichment ( 13 C-glucose/ 12 C-glucose) also was reduced in LIRKO mice relative to IR floxed and LIRFKO mice ( Fig. 3b ), indicating that the fraction of lactate derived from exogenous glucose is reduced in LIRKO mice and restored when FoxO1 expression is disrupted in the liver. These findings indicate that production of 13 C-lactate from 13 C-glucose (for example, by glycolysis) is impaired in LIRKO mice, consistent with a role for reduced disposal of exogenous glucose in the glucose intolerance of these animals. Since this defect is not present in LIRFKO mice, disruption of hepatic FoxO1 restores glucose tolerance to mice lacking hepatic IR, at least in part, by increasing glucose utilization. To determine whether changes in hepatic glucose metabolism might contribute to changes in glucose tolerance in LIRKO versus LIRFKO mice, we examined the expression of specific genes involved in glucose utilization and glucose production in livers collected 60 min following i.p. 13 C-glucose injection. Gene profiling studies indicated that glucokinase (Gck) expression is suppressed, and that the expression of glucose-6 phosphatase (G6Pase) and pyruvate dehydrogenase kinase 4 (PDK4) is increased in LIRKO mice compared with IR floxed and LIRFKO mice. As shown in Fig. 3c , quantitative real-time PCR studies demonstrated that the expression of Gck messenger RNA (mRNA) levels were ∼ 10-fold higher in both IR floxed and LIRFKO mice than in LIRKO mice, and western blotting confirmed that Gck protein levels were markedly reduced in LIRKO mice (insert) at this time point. This finding is important since Gck is a rate-limiting step in HGU, raising the possibility that (1) reduced HGU (owing in part to reduced Gck expression) contributes to glucose intolerance in LIRKO mice, and (2) the reversal of this defect in HGU contributes to the normalization of glucose homeostasis in LIRFKO mice. The expression of G6Pase, which dephosphorylates glucose-6 phosphate and thereby limits glucose utilization and promotes hepatic glucose secretion, was increased by approximately twofold in LIRKO versus IR floxed and LIRFKO mice ( Fig. 3c ). Similarly, the level of mRNA encoding PDK4, which phosphorylates pyruvate dehydrogenase and consequently inhibits the utilization of pyruvate for oxidative metabolism, was increased by approximately fourfold in LIRKO versus both IR floxed and LIRFKO mice. Together, these changes in gene expression also would be expected to reduce glucose utilization in LIRKO versus IR floxed and LIRFKO mice. We also examined the expression of phosphoenolpyruvate carboxykinase (PEPCK), a rate-limiting enzyme for gluconeogenesis that is regulated by insulin. As shown in Fig. 3c , levels of PEPCK mRNA were not increased in LIRKO versus IR floxed mice, indicating that differences in PEPCK expression did not contribute to impaired glucose tolerance in LIRKO versus IR floxed mice 60 min following i.p. glucose ( Fig. 3c ). PEPCK mRNA levels, however, were modestly reduced in LIRFKO versus IR floxed mice, suggesting that differences in PEPCK expression may contribute to improved glucose tolerance in LIRFKO mice. Euglycemic hyperinsulinemic clamp studies Previous studies have shown that that the ability of insulin to suppress HGP is impaired in LIRKO mice compared with floxed controls [16] . To determine whether disrupting FoxO1 restores the ability of insulin to suppress HGP in the absence of the hepatic IR, we performed euglycemic hyperinsulinemic clamp studies in LIRKO and LIRFKO mice. By design, euglycemia was maintained in both genotypes during hyperinsulinemia ( Fig. 4a ), but the glucose infusion rate (GIR) required to do so in LIRFKO mice was approximately twofold greater than in LIRKO mice ( Fig. 4b ), indicating markedly increased insulin sensitivity in the former group. This difference in GIR occurred despite the fact that insulin levels remained far higher in LIRKO than LIRFKO mice throughout the period from baseline to the end of the clamp procedure ( Fig. 4c ), providing additional evidence that loss of hepatic IR (in LIRKO mice) causes insulin resistance that is ameliorated by liver-specific deletion of FoxO1 (in LIRFKO mice). 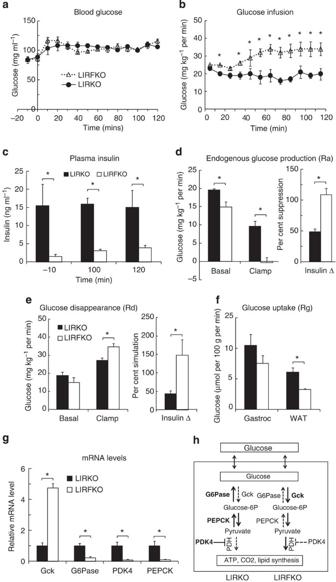Figure 4: Euglycemic hyperinsulinemic clamp. Circulating glucose levels (a), glucose infusion rates (b), insulin levels (c), endogenous glucose production (Ra) (d), total body glucose turnover rate (Rd) (e), glucose uptake (Rg) by gastrocnemius (gastroc) and white adipose tissue (WAT)(f), and hepatic gene expression at the end of the insulin clamp (g) in LIRKO (N=7) and LIRFKO (N=6) mice are shown as the mean and s.e.m. *P<0.05 LIRKO versus LIRFKO by two-tailed unpaired Student’st-test. (h) Hepatic glucose metabolism in LIRKO versus LIRFKO mice. Glucose is readily transported in and out of hepatocytes. In LIRFKO mice, glucose is phosphorylated by glucokinase (Gck) to form glucose-6 phosphate, which can be metabolized to form pyruvate, and then utilized for energy metabolism through the effect of pyruvate dehydrogense (PDH). Glucose utilization is limited in LIRKO liver due to reduced expression of Gck, increased expression of glucose-6 phosphatase (G6Pase), which dephosphorylates glucose-6 phosphate and promotes release of glucose by the liver, and increased expression of PDK4, which inhibits the ability to use pyruvate for energy metabolism. Pyruvate also can serve as a substrate for gluconeogenesis, and increased expression of PEPCK and the availability of pyruvate can both promote increased glucose production in LIRKO mice. In LIRFKO mice, glucose production is limited by reduced PEPCK expression and because pyruvate is able to be used for other purposes. Figure 4: Euglycemic hyperinsulinemic clamp. Circulating glucose levels ( a ), glucose infusion rates ( b ), insulin levels ( c ), endogenous glucose production (Ra) ( d ), total body glucose turnover rate (Rd) ( e ), glucose uptake (Rg) by gastrocnemius (gastroc) and white adipose tissue (WAT)( f ), and hepatic gene expression at the end of the insulin clamp ( g ) in LIRKO ( N= 7) and LIRFKO ( N= 6) mice are shown as the mean and s.e.m. * P <0.05 LIRKO versus LIRFKO by two-tailed unpaired Student’s t -test. ( h ) Hepatic glucose metabolism in LIRKO versus LIRFKO mice. Glucose is readily transported in and out of hepatocytes. In LIRFKO mice, glucose is phosphorylated by glucokinase (Gck) to form glucose-6 phosphate, which can be metabolized to form pyruvate, and then utilized for energy metabolism through the effect of pyruvate dehydrogense (PDH). Glucose utilization is limited in LIRKO liver due to reduced expression of Gck, increased expression of glucose-6 phosphatase (G6Pase), which dephosphorylates glucose-6 phosphate and promotes release of glucose by the liver, and increased expression of PDK4, which inhibits the ability to use pyruvate for energy metabolism. Pyruvate also can serve as a substrate for gluconeogenesis, and increased expression of PEPCK and the availability of pyruvate can both promote increased glucose production in LIRKO mice. In LIRFKO mice, glucose production is limited by reduced PEPCK expression and because pyruvate is able to be used for other purposes. Full size image Using isotope dilution with [3- 3 H]glucose, we demonstrated differences in the effects of insulin infusion on rates of both endogenous glucose production (endoRa, which largely reflects HGP; Fig. 4d ) and glucose disappearance ( Fig. 4e ) in LIRKO versus LIRFKO mice. In the basal state, the rate of HGP was ∼ 25% higher in LIRKO versus LIRFKO mice, supporting the concept that FoxO1 drives excessive HGP when hepatic IR signalling is disrupted. More importantly, hyperinsulinemia completely suppressed HGP in LIRFKO mice, but did so by only 50% in LIRKO mice. This result demonstrates that hepatic IR signalling is not required for the ability of systemic insulin to fully suppress HGP production when FoxO1 is disrupted in the liver and indicates the existence of an indirect (non-hepatic) mechanism(s) for control of HGP by insulin that is ineffective when FoxO1 is active in the liver as a result of hepatic IR deletion. While basal glucose disappearance (Rd) tended to be increased in LIRKO versus LIRFKO mice, consistent with differences in HGP, Rd was greater in LIRFKO mice compared with LIRKO at the end of the clamp ( Fig. 4e , left panel) and insulin was approximately three times more effective in stimulating Rd in LIRFKO mice ( ∼ 150% increase) compared with LIRKO mice (<50% increase; Fig. 4e , right panel). This difference in Rd (LIRFKO>LIRKO) did not appear to be due to differences in glucose utilization in other insulin-responsive tissues, since glucose uptake, measured by infusing labelled 2-deoxyglucose at the end of the insulin clamp, was higher in white adipose tissue (WAT) and also tended to be increased gastrocnemius in LIRKO versus LIRFKO mice ( Fig. 4f ). The apparent discrepancy between insulin-stimulated Rd (LIRFKO>LIRKO) and glucose uptake in WAT and skeletal muscle (LIRKO>LIRFKO) suggested the possibility that differences in HGU (which cannot be measured with 2-deoxglucose due to the presence of G6Pase) may contribute to differences in Rd, and studies of hepatic gene expression support this concept. As shown in Fig. 4f , hepatic expression of Gck was increased by approximately fivefold in LIRFKO versus LIRKO mice at the end of the clamp period, while G6Pase and PDK4 were suppressed by ∼ 90% in LIRFKO compared with LIRKO mice. These differences in Gck, G6Pase and PDK4 would all serve to increase glucose utilization in the liver of LIRFKO mice relative to LIRKO ( Fig. 4f ). Hepatic PEPCK expression also was strongly suppressed in LIRFKO versus LIRKO mice at the end of the clamp, and differences in both PEPCK and G6pase expression would serve to reduce HGP in LIRFKO mice compared with LIRKO. These results indicate that changes in hepatic Gck, G6Pase, PDK4 and PEPCK gene expression contribute to differences in insulin-regulated HGP and glucose utilization in LIRFKO versus LIRKO mice ( Fig. 4f ). Nutritional regulation of hepatic gene expression To further characterize the regulation of hepatic gene expression during fasting and 6 h after refeeding, when effects of nutrient availability and insulin levels on hepatic gene expression are apparent [18] , mice were fasted overnight for 18 h and then either refed or allowed to continue fasting until sacrifice 6 h later. As expected, circulating levels of corticosterone were elevated during fasting relative to the re-fed condition, and this response did not differ between genotypes ( Fig. 5a ). Fasting serum levels of free fatty acids were somewhat lower in LIRKO mice than either IR floxed or LIRFKO mice ( Fig. 5b ), presumably reflecting the anti-lipolytic effect of increased insulin levels in LIRKO mice ( Fig. 2b ). Nevertheless, levels of free fatty levels were suppressed to a similar extent in each genotype following refeeding. These results indicate that the systemic response to refeeding, including changes in circulating levels of corticosterone and free fatty acids is largely intact in LIRKO mice. 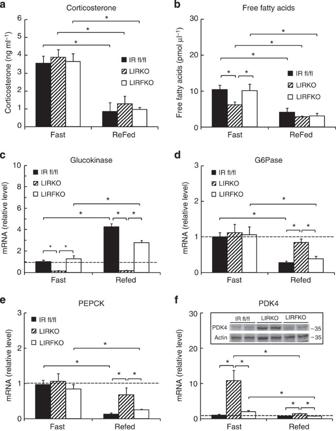Figure 5: Nutritional regulation of gene expression. IR floxed, LIRKO and LIRFKO mice were fasted overnight for 18h and then refed or allowed to continue fasting until they were killed 6h later. Cervical blood was collected for analysis of serum levels of glucose and insulin (Fig. 2) and for levels of (a) corticosterone (N=8, 4 and 6 fasting, and 4, 5 and 4 refed IR floxed, LIRKO and LIRFKO mice, respectively), and (b) free fatty acids (N=8, 6 and 6 fasting, and 5, 6 and 6 refed IR floxed, LIRKO and LIRFKO mice, respectively). (c–f) mRNA levels for (c) glucokinase, (d) glucose-6 phosphatase, (e) PEPCK and (f) PDK4 were measured by quantitative PCR in fasting and refed IR floxed (N=5 fasting, 6 refed), LIRKO (N=7 fasting, 4 refed) and LIRKO (N=6 fasting, 5 refed) mice. Disruption of FoxO1 restores the ability of refeeding to regulate the expression of glucokinase, G6Pase and PEPCK in the liver despite the absence of hepatic IR in LIRFKO mice. Results are presented as the mean and s.e.m. *P<0.5 by one way analysis of variance and Fisher’spost-hoctest. Figure 5: Nutritional regulation of gene expression. IR floxed, LIRKO and LIRFKO mice were fasted overnight for 18h and then refed or allowed to continue fasting until they were killed 6h later. Cervical blood was collected for analysis of serum levels of glucose and insulin ( Fig. 2 ) and for levels of ( a ) corticosterone ( N= 8, 4 and 6 fasting, and 4, 5 and 4 refed IR floxed, LIRKO and LIRFKO mice, respectively), and ( b ) free fatty acids ( N= 8, 6 and 6 fasting, and 5, 6 and 6 refed IR floxed, LIRKO and LIRFKO mice, respectively). ( c – f ) mRNA levels for ( c ) glucokinase, ( d ) glucose-6 phosphatase, ( e ) PEPCK and ( f ) PDK4 were measured by quantitative PCR in fasting and refed IR floxed ( N= 5 fasting, 6 refed), LIRKO ( N= 7 fasting, 4 refed) and LIRKO ( N= 6 fasting, 5 refed) mice. Disruption of FoxO1 restores the ability of refeeding to regulate the expression of glucokinase, G6Pase and PEPCK in the liver despite the absence of hepatic IR in LIRFKO mice. Results are presented as the mean and s.e.m. * P <0.5 by one way analysis of variance and Fisher’s post-hoc test. Full size image Gck expression was reduced in fasting LIRKO versus IR floxed mice and this effect was reversed in LIRFKO mice ( Fig. 5c ). Thus, loss of hepatic IR signalling reduces Gck expression even under fasting conditions when insulin levels are low, and FoxO1 is required for this effect. Hepatic Gck mRNA levels increased by approximately fourfold after refeeding in IR floxed mice, but did not increase in LIRKO mice. Disruption of FoxO1 partially rescued the ability of refeeding to upregulate Gck expression in mice lacking hepatic IR (approximately twofold increase in refed versus fasting LIRFKO). These results demonstrate that hepatic IR signalling is required for the induction of Gck expression after refeeding, and genetic deletion of FoxO1 partially abrogates this requirement for insulin signalling in the liver. In contrast to Gck, G6Pase expression was similar in fasted IR floxed, LIRKO and LIRFKO mice ( Fig. 5d ), indicating that neither hepatic IR signalling nor FoxO1 is required for normal G6Pase expression in the fasted state. As expected, refeeding reduced G6Pase expression in IR floxed mice, but this effect was not observed in LIRKO mice, indicating that hepatic IR signalling is required for suppression of G6Pase expression in response to refeeding. In contrast, G6Pase expression was suppressed normally by refeeding in LIRFKO mice, demonstrating that disrupting the function of FoxO1 restores the ability of refeeding to suppress the expression of G6Pase in the liver in the absence of hepatic IR signalling. Like G6Pase, liver PEPCK mRNA levels were comparable in IR floxed, LIRKO and LIRFKO mice during fasting ( Fig. 5e ), indicating that during fasting, regulation of PEPCK expression is largely independent of hepatic IR signalling and FoxO1. Also like G6Pase, after refeeding PEPCK gene expression was reduced in IR floxed mice and LIRFKO mice but not in LIRKO mice, indicating that hepatic IR signalling is required for suppression of PEPCK expression by refeeding, and that deletion of FoxO1 restores the ability of refeeding to lower hepatic PEPCK expression when hepatic IR signalling is disrupted. Hepatic PDK4 expression was increased by >10-fold in LIRKO versus IR floxed mice ( Fig. 5f ), indicating that hepatic IR signalling plays an important role in limiting PDK4 expression during fasting, even though insulin levels are low. PDK4 mRNA levels were restored to control levels in LIRFKO mice, indicating that FoxO1 is important for the induction of PDK4 expression when hepatic insulin signalling is disrupted, consistent with previous studies [19] . PDK4 expression was strongly suppressed by refeeding in LIRKO mice, perhaps reflecting changes in circulating levels of glucocorticoids [20] . Nevertheless, PDK4 expression remained approximately twofold higher in LIRKO versus both IR floxed and LIRFKO mice after refeeding, indicating that disruption of FoxO1 restores the ability of refeeding to fully suppress PDK4 expression in the absence of hepatic IR signalling. These results indicate that disrupting the function of FoxO1 in the liver is sufficient to restore effects of food intake on Gck, G6Pase, PEPCK and PDK4 gene expression in the absence of hepatic IR signalling, presumably due, at least in part, to extrahepatic effects of insulin and possibly other nutrient-mediated effects on hepatic gene expression. In this study, we generated LIRFKO mice to investigate the role of hepatic IR-FoxO1 signalling in whole body and liver glucose homeostasis. This approach yielded several fundamental insights. Most notably, disrupting FoxO1 in the liver fully restored glucose tolerance, glucose lowering effects of insulin and the ability of insulin to fully suppress HGP despite the absence of the hepatic IR. In contrast, disrupting FoxO1 had limited effect on hepatic glycogen content, indicating that changes in glycogen metabolism are not a major factor in restoring glucose homeostasis in LIRFKO versus LIRKO mice. Perhaps most importantly, our data indicate that, in addition to its direct action on hepatocytes, insulin also can inhibit HGP via an indirect pathway (or pathways) that functions independently of the hepatic IR, and that suppression of FoxO1 activity downstream from the IR appears to be required for this indirect pathway to be effective. It is interesting to note that in previous studies disrupting FoxO1 in the liver of mice with intact IR function had only a modest effect on fasting glucose levels and glucose tolerance, and that knocking out multiple hepatic FoxOs was necessary to strongly perturb glucose homeostasis in animals with intact hepatic IR function [3] , [4] . This contrasts sharply with the dramatic effect on glucose homeostasis that results when FoxO1 is deleted in the liver of mice lacking hepatic IRs. While multiple FoxO proteins in the liver may contribute to the regulation of glucose homeostasis under normal conditions, our results indicate that FoxO1 is a critical mediator of impaired glucose homeostasis in the setting of hepatic insulin resistance. Previous studies also have shown that disrupting FoxO1 in the liver restores glucose tolerance [12] , [13] and the ability of insulin to suppress HGP [13] in mice in which downstream mediators of insulin signalling have been genetically disrupted, but did not address whether insulin action in this setting is mediated at a non-hepatic site or via other signalling pathways downstream of the hepatic IR [13] . This study establishes that downstream effects of hepatic IR-mediated signalling are not required for insulin regulation of HGP in the absence of hepatic FoxO1. Related studies by Titchenell et al. [21] confirm that the ability of insulin to suppress gluconeogenic gene expression is disrupted in isolated hepatocytes from LIRKO and LIRFKO mice, providing additional support for the concept that cell non-autonomous effects of insulin are required to restore insulin regulation of HGP in LIRFKO mice. Further, we find that blocking extrahepatic IR-mediated effects of insulin with the IR specific inhibitor S961 disrupts glucose tolerance and glucose lowering effects of insulin in LIRFKO mice. Together, these studies support the concept that indirect effects that are mediated through extrahepatic targets of insulin action are required to maintain glucose homeostasis and sufficient to regulate HGP when both the IR and FoxO1 are disrupted in the liver. That insulin can regulate HGP via an indirect pathway was suggested 17 years ago [22] , but its physiological relevance has remained uncertain, and a counterargument has been made that the action of insulin directly on hepatocytes is the primary mechanism through which insulin controls of HGP [23] . Although direct hepatic effects of insulin may be sufficient to inhibit HGP, our results indicate that they are not required in vivo when effects of FoxO1 in the liver are disrupted. The original report of increased HGP and glucose intolerance in LIRKO mice [16] was taken as evidence that normal glucose homeostasis requires intact liver insulin signalling and our study supports this concept. However, the current data also suggest that this conclusion must be modified to recognize that (a) the disruption of glucose homeostasis in LIRKO mice is FoxO1 dependent, and that (b) when hepatic FoxO1 function is disrupted indirect effects of insulin involving extrahepatic targets of insulin also are sufficient to regulate HGP. In addition to its role in mediating effects of insulin on HGP, we find that hepatic FoxO1 also contributes to the regulation of glucose utilization. Studies with 13 C-glucose showed that glucose disposal is reduced in LIRKO mice, and disruption of FoxO1 in the liver reversed this effect. Similarly, insulin clamp studies showed that insulin-stimulated glucose disappearance was impaired in LIRKO relative to LIRFKO mice. In both cases, gene expression studies indicate that, in addition to its effects on HGP, hepatic FoxO1 also promotes glucose intolerance, at least in part, by reducing HGU, reflecting changes in the expression of Gck, G6Pase and PDK4 in the liver. Studies in transgenic and knockout mice support the concept that FoxO proteins exert significant effects on glucose metabolism due, at least in part, to changes in the expression of Gck [2] , [5] , [24] , a master regulator of hepatic glucose metabolism. This study provides direct evidence that FoxO1 plays a major role in regulating Gck expression downstream from the hepatic IR in vivo . Additional studies are needed to determine why suppressing FoxO1 in the liver is required for extrahepatic effects of insulin to be effective in regulating hepatic glucose metabolism. As suggested in Fig. 6 , it may be necessary for insulin to suppress the function of hepatic FoxO1 for insulin-regulated extrahepatic signals (for example, changes in levels of free fatty acids [25] , [26] ) to be effective in regulating hepatic glucose metabolism. Alternatively, FoxO1-regulated factors that are produced by the liver (‘hepatokines’) may impair the ability of insulin to act on extrahepatic tissues that generate signals involved in regulating HGP. Related to this concept, recent studies suggest that other circulating factors produced by the liver promote beta cell proliferation and islet hyperplasia in LIRKO mice [27] , and our finding that knocking out FoxO1 in the liver prevents islet hyperplasia in the setting of hepatic insulin resistance ( Fig. 2e ) suggests that these as yet unidentified hepatokines and others may be regulated by FoxO1. 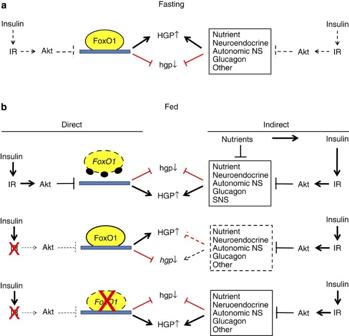Figure 6: Regulation of hepatic glucose production (HGP) and hepatic utilization (HGU) by insulin and FoxO1. (a) Fasting. In fasting, insulin levels are low and FoxO1 is transcriptionally active in the liver where it exerts effects that promote HGP and suppress HGU. At the same time, extrahepatic signals (for example, increased levels of free fatty acids, glucagon and input from the neuroendocrine and autonomic nervous systems) also promote increased HGP and decreased HGU. (b) Fed. Top panel. After refeeding, increased insulin signalling in the liver activates Akt, which phosphorylates and disrupts effects of FoxO1 on gene expression and hepatic glucose production (HGP) and utilization (HGU). At the same time, insulin and nutrients exert effects on extrahepatic signals that also contribute to the reduction in HGP and increase in HGU. Middle panel. In the setting of hepatic insulin resistance, Akt is not activated and hepatic FoxO1 continues to promote increased HGP and reduced HGU. Extrahepatic signals are no longer effective in regulating HGP and HGU due to continued activity of FoxO1 in the liver. Bottom panel. Disruption of FoxO1 in the liver restores the ability of extrahepatic signals to regulate HGP and HGU in response to fasting and refeeding. Figure 6: Regulation of hepatic glucose production (HGP) and hepatic utilization (HGU) by insulin and FoxO1. ( a ) Fasting. In fasting, insulin levels are low and FoxO1 is transcriptionally active in the liver where it exerts effects that promote HGP and suppress HGU. At the same time, extrahepatic signals (for example, increased levels of free fatty acids, glucagon and input from the neuroendocrine and autonomic nervous systems) also promote increased HGP and decreased HGU. ( b ) Fed. Top panel. After refeeding, increased insulin signalling in the liver activates Akt, which phosphorylates and disrupts effects of FoxO1 on gene expression and hepatic glucose production (HGP) and utilization (HGU). At the same time, insulin and nutrients exert effects on extrahepatic signals that also contribute to the reduction in HGP and increase in HGU. Middle panel. In the setting of hepatic insulin resistance, Akt is not activated and hepatic FoxO1 continues to promote increased HGP and reduced HGU. Extrahepatic signals are no longer effective in regulating HGP and HGU due to continued activity of FoxO1 in the liver. Bottom panel. Disruption of FoxO1 in the liver restores the ability of extrahepatic signals to regulate HGP and HGU in response to fasting and refeeding. Full size image Together, these studies highlight the central and complex role hepatic FoxO1 plays in regulating glucose metabolism in response to insulin. In addition to mediating direct effects of insulin on hepatic gene expression and metabolism, suppression of FoxO1 function within the liver also appears to be critical for the ability of insulin to regulate hepatic glucose metabolism and maintain normal glucose homeostasis through IR-mediated effects on extrahepatic tissues. Based on these findings, targeting FoxO1 in the liver may provide an effective strategy for the treatment of diabetes mellitus in patients with hepatic insulin resistance by enabling the ability of extrahepatic effects of insulin to maintain glucose homeostasis. Generation of knockout mice and in vivo studies The institutional animal care and use committees of the Jesse Brown VA Medical Center and Vanderbilt University Medical School approved all animal studies. Albumin-Cre (Jackson Laboratories), FoxO1 floxed [28] (from Ron DePinho, Dana Farber Cancer Institute) and IR floxed [16] mice were crossed to create IR floxed, IR fl/fl -FoxO1 fl/fl (IR/FoxO floxed) and LIRKO and LIRFKO mice on a mixed (C57Bl/6-FVB/N) background. Male mice were used to limit variability. Mice were housed on a 0600:1800 hours light/dark cycle. Body composition of 8-week-old mice was determined by NMR (LF50 BCA-Analyser, Bruker). 12 C- and 13 C-glucose tolerance tests were performed following an 18 h overnight fast in 9–10-week-old mice by i.p. injection of dextrose ( 12 C-glucose) or D-[UL- 13 C 6 ]-glucose (13C-glucose; 2 g/kg), with glucose levels monitored serially by tail vein bleed at time=0, 15, 30, 60 and 90 min using a One Touch glucose meter (Lifescan). In studies with 13 C-glucose, mice were killed at 60 min to collect plasma and liver for subsequent analysis. In a subset of mice, an insulin tolerance test was performed 1 week later following a 4 h fast by i.p. injection with 1 U kg −1 human insulin (Humulin, Lilly) and monitoring of glucose levels as before. In some studies, mice were treated with S961 (Novo Nordisk; 1.1 nmol per mouse) or phosphate-buffered saline (PBS) s.c. alone 30 min prior to glucose or insulin tolerance testing. For fasting/refeeding studies, 12-week-old mice were fasted overnight (18 h) and then either refed or continued fasting until sacrifice 6 h later. Cervical blood was collected and the liver was removed, weighed, and then frozen in liquid N2 and stored at −80 °C for analysis. Hyperinsulinemic euglycemic clamps Insulin clamp studies were performed in 16–20-week-old male mice at the Vanderbilt University Mouse Metabolic Phenotyping Center ( www.mc.vanderbilt.edu/mmpc ). Carotid artery and jugular vein catheters were implanted in mice 5–6 days before the insulin clamp [29] , [30] . Insulin clamps were performed on 5-h fasted mice. [3- 3 H]glucose infusions were primed (2.4 μCi) and then continued for a 90-min equilibration period (0.04 μCi min −1 ) prior to a 2-h clamp period (0.12 μCi min −1 ). [3- 3 H]glucose also was mixed with the glucose infused i.v. to maintain both glucose concentrations and specific activity constant during the 4 mU kg −1 min −1 insulin infusion. Baseline blood glucose and plasma insulin levels were determined in samples collected at −15 and −5 min. Insulin infusion (4 mU kg −1 min −1 ) was started at t= 0 and continued for 165 min. Blood glucose, monitored every 10 min, was clamped at 150–160 mg dl −1 by varying the GIR. Mice received 5 μl min −1 heparinized saline-washed erythrocytes to maintain a stable haematocrit. Blood [3- 3 H]glucose was determined at 80–120 min and insulin levels were determined at t =100 and 120 min. 13 μCi of 2-[ 14 C]deoxyglucose ([ 14 C]2DG) was administered as an i.v. bolus 35 min before the end of the study to measure glucose disposal (Rg). Plasma insulin was determined by ELISA and radioactivity of [3- 3 H]glucose, ciculating [ 14 C]2DG and tissue [ 14 C]2DG-6-phosphate were determined by liquid scintillation counting. Glucose appearance ( R a ) and disappearance ( R d ) rates were determined using non-steady-state equations [31] and endogenous glucose production ( R a ) was determined by subtracting the GIR from total R a . Histochemistry and electron microscopy Liver and pancreas were fixed in Z-fix (Anatech) for 18 h at 4 °C, rinsed in PBS and stored in 70% ethanol prior to processing and embedding in paraffin in the University of Illinois Histology Core. Tissues were stained with haematoxylin and eosin prior to scanning at × 200 with an Aperio Scanscope CS. Sections (4-μm-thick) of pancreata were probed with anti-insulin antibody prior to scanning at × 200 with an Aperio Scanscope CS and quantification of total tissue and islet cross-sectional area using ImageScope software (Aperio). For transmission electron microscopy studies, 1–2-mm thick liver sections were fixed in 2.5% glutaraldehyde, 2% paraformaldehyde in PBS overnight at 4 °C prior to imaging with a JEOL JEM 1011 transmission electron microscope (Peabody) at 80 kV fitted with a side mount AMT digital camera (Advanced Microscopy Techniques) [19] . Circulating levels of insulin, C-peptide and glucose and lactate isotopomers Serum insulin and C-peptide levels were measured by ELISA kits as per the manufacturer’s instructions (ALPCO). Plasma 12 C- and 13 C-glucose levels were measured by liquid chromatography/mass spectroscopy. Liquid chromatography was performed with Luna NH2 HILIC column (Phenomenex) using an Agilent 1200 chromatography system (Agilent technologies, CA), Luna NH2 HILIC (hydrophilic interaction liquid chromatography) column and mass spectrometry was performed using an Agilent 6520 series Quadrupole-Time-of-flight mass spectrometer (Agilent technologies) in the University of Michigan Regional Comprehensive Metabolomics Resource Core ( http://mrc2.umich.edu ). For analysis of lactate, samples were derivatized and analysed by gas chromatography/mass spectroscopy with an Agilent 7890 with 5975 MSD (Agilent Technology) using a DB-5MS column. All data was processed by MassHunter workstation software, version B.06. Gene expression and western blotting studies Total hepatic RNA was prepared using RNeasy kits (Qiagen). Gene array studies and data analysis were performed in the University of Illinois Functional Genomics Unit using Agilent Mouse 4 × 44 K V2 microarrays and a false discovery rate of <0.05 was used to identify differentially expressed genes between genotypes. Levels of specific transcripts were quantified by real-time PCR (MyiQ, BioRad) using Syber Green on a MyiQ detection system (BioRad) using specific primers for Gck (forward—5′-TATGAAGACCGCCAATGTGA-3′; reverse—5′-TTTCCGCCAATGATCTTTTC-3′), G6Pase (forward—5′-ATCCGGGGCATCTACAATG; reverse—5′-TGGCAAAGGGTGTAGTGTCA-3′), PEPCK (forward—5′-TGTTTACTGGGAAGGCATCG-3′; reverse—5′-AGGTCTACGGCCACCAAAG-3′), IGF-1R (forward—5′-AGGAATGTGGGGACCTGTGT-3′; reverse—5′-GTGGCAGCACTCGTTGTTCT-3′), IR (forward—5′-CCCCACCCTTTGAGTCTGAT-3′; reverse—5′-CTG TCACATTCCCCACCTCT-3′), PDK-4 (forward—5′-GCCTTGGGAGAAATGTGTGT; reverse—5′-CACTGGCTTTTTGAGTGCAA-3′) and results were adjusted for differences in the expression of mouse TATA binding protein (mTBP) (forward—5′-ACCCTTCACCAATGACTCCTATG-3′: reverse—5′-ATGATGACTGCAGCAAATCGC-3′) to correct for internal variances. For western blotting, hepatic lysates were prepared with T-PER (Thermo Scientific) in the presence of protease and phosphatase inhibitors and protein content was quantified prior to separation by Laemmli gel electrophoresis and electrotransfer for analysis using specific antibodies for the IR beta subunit (Cat No. 3025, 1:1,000 dilution), total Akt (Cat No. 9272, 1:1,000 dilution), phospho-ser473 Akt (Cat No. 9270, 1:1,000 dilution), total FoxO1 (Cat No. 2880, 1:1,000 dilution), phospho-ser256 FoxO1 (Cat No. 9461, 1:500 dilution) and actin (Cat No. 4970, 1:1,000 dilution) from Cell Signaling or antibody against Gck (Santa Cruz, Cat No. 7908, 1:200 dilution) or PDK4 (provided by Robert Harris [32] , 1:500 dilution). Full length western blots are shown in Supplementary Fig. 1 . Statistics Results are presented as the mean and s.e.m. and 5–12 mice were studied per group unless otherwise stated. Statistical significance of differences between groups was determined by one-way analysis of variance and Fisher’s least significant difference test unless otherwise stated. Accession Codes: Gene expression data have been deposited in the gene expression omnibus (GEO) database repository under accession code GSE59885YYY . How to cite this article: O-Sullivan, I. et al. FoxO1 integrates direct and indirect effects of insulin on hepatic glucose production and glucose utilization. Nat. Commun. 6:7079 doi: 10.1038/ncomms8079 (2015).